Information–theoretic implications of quantum causal structures It is a relatively new insight of classical statistics that empirical data can contain information about causation rather than mere correlation. First algorithms have been proposed that are capable of testing whether a presumed causal relationship is compatible with an observed distribution. However, no systematic method is known for treating such problems in a way that generalizes to quantum systems. Here, we describe a general algorithm for computing information–theoretic constraints on the correlations that can arise from a given causal structure, where we allow for quantum systems as well as classical random variables. The general technique is applied to two relevant cases: first, we show that the principle of information causality appears naturally in our framework and go on to generalize and strengthen it. Second, we derive bounds on the correlations that can occur in a networked architecture, where a set of few-body quantum systems is distributed among some parties. A causal structure for a set of classical variables is a graph, where every variable is associated with a node and a directed edge denotes functional dependence. Such a causal model offers a means of explaining dependencies between variables, by specifying the process that gave rise to them. More formally, variables X 1 , …, X n form a Bayesian network with respect to a directed, acyclic graph (commonly abbreviated DAG), if every variable X i depends only on its graph–theoretic parents PA i . This is the case [1] , [2] if and only if the distribution factorizes as in One can ask the following fundamental question: given a subset of variables, which correlations between them are compatible with a given causal structure? In this work, we measure ‘correlations’ in terms of the collection of joint entropies of the variables, which we allow to be quantum systems as well as classical random variables (a precise definition will be given below). This problem appears in several contexts. In the young field of causal inference, the goal is to learn causal dependencies from empirical data [1] , [2] . If observed correlations are incompatible with a presumed causal structure, it can be discarded as a possible model. This is close to the reasoning employed in Bell’s theorem [3] —a connection that is increasingly appreciated among quantum physicists [4] , [5] , [6] , [7] , [8] , [9] , [10] . In the context of communication theory, these joint entropies describe the capacities that can be achieved in network-coding protocols [11] . In this work, we are interested in quantum generalizations of causal structures. Nodes are now allowed to represent either quantum or classical systems, and edges are quantum operations. An important conceptual difference to the purely classical set-up is rooted in the fact that quantum operations disturb their input. Put differently, quantum mechanics does not assign a joint state to the input and the output of an operation. Therefore, there is in general no analogue to (1), that is, a global density operator for all nodes in a quantum causal structure cannot be defined. However, if we pick a set of nodes that do coexist (for example, because they are classical, or because they are created at the same instance of time, that is, they do have a joint density operator), then we can again ask: which joint entropies of coexisting nodes can result from a given quantum causal structure? Here, we answer this question by introducing a universal framework that generalizes previous results on the classical case [6] , [7] , [12] , [13] , [14] . This framework’s versatility and practical relevance can be illustrated with two examples. In the context of distributed quantum architectures [15] , [16] , [17] , [18] , [19] , the framework can be employed to systematically compute limits on the correlations that are imposed solely by the topology of the networks. The machinery can also be used to generalize and strengthen information causality (IC) [20] , a principle that may explain the ‘degree of non-locality’ exhibited by quantum mechanics. The details, along with more examples including dense coding schemes [21] , are presented in the main text. Quantum causal structures Informally, a quantum causal structure specifies the functional dependency between a collection of quantum systems and classical variables. We find it helpful to employ a graphical notation, where we aim to closely follow the conventions of classical graphical models [1] , [2] . There are two basic building blocks: root nodes are labelled by a set of quantum systems and represent a density operator for these systems The second type is given by nodes with incoming edges. Again, both the edges and the node carry the labels of quantum systems. Such symbols represent a quantum operation (completely positive, trace-preserving (CPTP) map) from the systems associated with the edges to the ones associated with the node: These blocks may be combined: a node containing a system X can be connected to an edge with the same label. The interpretation is, of course, that X serves as the input to the associated operation. For example, says that the state of system C is the result of applying an operation Φ AB→C to a product state on AB. To avoid ambiguities, we will never use the same label in two different nodes (in particular, we always assume that the output systems of an operation are distinct from the input systems). For a more involved example, note that Fig. 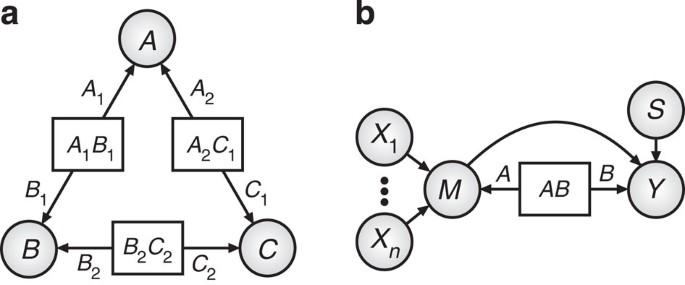Figure 1: Causal structures. (a) An example of distributed architecture involving bipartite entangled states. Each of the underlying quantum states can connect at most two of the observable variables, which implies a non-trivial monogamy of correlations as captured in (12). (b) The quantum causal structure associated with the information causality principle. 1a gives a fairly readable representation of the following cumbersome algebraic statement: Figure 1: Causal structures. ( a ) An example of distributed architecture involving bipartite entangled states. Each of the underlying quantum states can connect at most two of the observable variables, which implies a non-trivial monogamy of correlations as captured in (12). ( b ) The quantum causal structure associated with the information causality principle. Full size image (where the operation defined in the first line is acting on the state defined in the second line). The graphical representation does not indicate which input state or which operation to employ. We suppress this information, because we will be interested only in constraints on the resulting correlations that are implied by the topology of the interactions alone, regardless of the choice of states and maps. We denote the labels of classical variables (equivalently, quantum systems described by states that are diagonal in a given basis) in circles, as opposed to the rectangles we use for quantum systems. In principle, classical variables could have >1 outgoing edge. Of course, the no-cloning principle precludes a quantum system being used as the input to two different operations. Moreover, only graphs that are free of cyclic dependencies can be interpreted as specifying a causal structure. Thus, as is the case in classical Bayesian networks, every quantum causal structure is associated with a DAG. We note that graphical notations for quantum processes have been used frequently before. The most popular graphical calculus is probably the gate model of quantum computation [22] , where, directly opposite to our conventions, operations are nodes and systems are edges. That is also the case in the recently introduced generalized Bayesian networks in ref. 9 . There, the authors even allow for post-quantum resources. Quantum communication scenarios are often visualized the same way we employ here [23] . We have noted in the introduction that a classical Bayesian network not only defines the functional dependencies between random variables, but also provides a structural formula (1) for the joint distribution of all variables in the graph. Again, such a joint state for all systems that appear in a quantum causal structure is not in general defined. However, other authors have considered quantum versions of distributions that factor as in (1) and have developed graphical notations to this end. Well-known examples include the related constructions that go by the name of finitely correlated states, matrix–product states, tree–tensor networks or projected entangled pairs states (a highly incomplete set of starting points to the literature is given in refs 24 , 25 , 26 ). Also, certain definitions of quantum Bayesian networks [27] , [28] fall into that class. Entropic description of quantum causal structures The entropic description of classical-quantum DAGs can be seen as a generalization of the framework for the case of purely classical variables [6] , [7] , [12] , [13] , [14] that consists of three main steps. Consider a classical DAG consisting of n variables and a subset of them that are observable. In step 1, one needs to construct a description of the unconstrained Shannon cone. As we will see below, this means enumerating all elementary inequalities that entropies of n variables must respect, regardless of their causal relations. In step 2, the causal constraints must be added, which corresponds to listing all conditional independence relations implied by the DAG. In step 3, a marginalization is performed, that is, because some of the variables may not be observable, these need to be eliminated from our description. The final result of this three-step programme is the description of the marginal entropic constraints implied by the model under investigation. To further understand the meaning of these steps and how they need to be modified to cope with quantum causal structures, in the following we briefly discuss each of them. To begin with, we denote the set of indices of the random variables by [ n ]={1, …, n } and its power set (that is, the set of subsets) by 2 [ n ] . For every subset S ε2 [ n ] of indices, let X S be the random vector ( X i ) i ε S and denote by H ( S ):= H ( X S ) the associated entropy vector (for some, still unspecified entropy function H ). Entropy is then a (partial) function H :2 [ n ] → , S ↦ H ( S ) on the power set. Note that as entropies must fulfil some constraints, not all entropy vectors are possible. That is, given the linear space of all set functions denoted by R n and a function h ε R n the region of vectors in R n that correspond to entropies is given by Clearly, this region will depend on the chosen entropy function. For classical variables, H is chosen to be the Shannon entropy given by . In this case, an outer approximation to the associated entropy region has been studied extensively in information theory, the so-called Shannon cone Γ n (ref. 11 ), which is the basis of the entropic approach in classical causal inference [14] . The Shannon cone is the polyhedral closed convex cone of set functions h that respect two elementary inequalities, known as polymatroidal axioms. The first relation is the sub-modularity (also known as strong subadditivity) condition, which is equivalent to the positivity of the conditional mutual information, for example, I ( A : B | C )= H ( A , C )+ H ( B , C )− H ( A , B , C )− H ( C )≥0. The second inequality—nown as monotonicity—is equivalent to the positivity of the conditional entropy, for example, H ( A | B )= H ( A , B )− H ( B )≥0. Therefore, the first step of the algorithm corresponds to listing all these elementary inequalities. The elementary inequalities discussed above encode the constraints that the entropies of any set of classical variables are subject to, regardless of their causal relations. Therefore, in the second step of the algorithm we need to list the causal relationships between the variables. These are encoded in the conditional independences (CIs) implied by the graph and can be algorithmically enumerated using the so-called d-separation criterion [1] . Therefore, if one further demands that classical random variables are a Bayesian network with respect to some given DAG, their entropies will also fulfil the additional CI relations implied by the graph. The CIs, relations of the type p ( x , y | z )= p ( x | z ) p ( y | z ) that defines nonlinear constraints in terms of probabilities, are equivalent to homogeneous linear constraints on the level of entropies, for example, I ( X : Y | Z )=0. Finally, we are interested in situations where not all joint distributions are accessible. Most commonly, this is because the variables of a DAG can be divided into observable and not observable ones (for example, the underlying quantum states in Fig. 1 ). Given the set of observable variables, in the classical case, it is natural to assume that any subset of them can be jointly observed. However, in quantum mechanics that situation is more subtle. For example, position Q and momentum P of a particle are individually measurable, however, there is no way to consistently assign a joint distribution to both position and momentum of the same particle [3] . That is while H ( Q ) and H ( P ) are part of the entropic description of classical-quantum DAGs, joint terms such as H ( Q , P ) cannot be part of it. This motivates the following definition: given a set of variables X 1 , …, X n contained in a DAG, a marginal scenario is the collection of those subsets of X 1 , …, X n that are assumed to be jointly measurable. Given the inequality description of the DAG and the marginal scenario under consideration, the third and last step of the algorithm consists of eliminating from this inequality description the variables that are not observable, that is the variables that are not contained in . This is achieved, for example, via a Fourier–Motzkin (FM) elimination (see Methods for further details). We now turn our attention to the generalization of the algorithm to include quantum systems, that are described in terms of the quantum analogue of the Shannon entropy, the von Neumann entropy H (ϱ A,B )=−Tr (ϱ A,B log ϱ A,B ). In the first step of the algorithm there are two differences. First, while quantum systems respect sub-modularity, the von Neumann entropy fails to comply with monotonicity. In this case, one needs to resort to the weak version of the monotonicity inequality (for example, H (ϱ A )+ H (ϱ B )≤ H (ϱ AC )+ H (ϱ BC )), a constraint that is fulfilled by the von Neumann entropy. Note, however, that for sets consisting of both classical and quantum systems, monotonicity may still hold. That is because the uncertainty about a classical variable A cannot be negative, even if we condition on an arbitrary quantum system ϱ, following then that H ( A |ϱ)≥0 (ref. 29 ). Furthermore, for a classical variable A , the entropy H ( A ) reduces to the Shannon entropy [30] . The second difference is the fact that measurements, or more generally CPTP maps, on a quantum state will generally destroy/disturb the state. To illustrate that, consider the classical-quantum DAG in Fig. 1 . Consider the classical and observable variable A . It can without loss of generality be considered a deterministic function of its parents and , as any additional local parent can be absorbed in one of the latter. For the variable A to assume a definite outcome, a joint CPTP map is applied to both parents and that will in general disturb these variables. The random variable A does not coexist with quantum systems A 1 and A 2 . Therefore, no entropy can be associated to these variables simultaneously, that is, H ( A , A 1 , A 2 ) cannot be part of the entropic description of the classical-quantum DAG. As a result of that, only elementary inequalities involving coexisting variables can be listed in step 1. Classically, this problem does not arise as the underlying classical hidden variables could be accessed without disturbing them. In the second step of the algorithm, we need to list all the causal relations as encoded in CIs implied by the graph. All the classical CIs (that is, following from the d-separation criterion) that involve coexisting variables also hold for the quantum causal structures considered here [9] . However, some classically valid CIs may, in the quantum case, involve non-coexisting variables and therefore are not valid for quantum systems. As an example, consider the DAG in Fig. 1b . For the classical analogue of this DAG it follows, for example, that I ( A : B | A 1 , A 2 , B 1 , B 2 ). This relation states that the correlations between A and B should be screened off conditioned on their common ancestor. Because this CI involves a term such as H ( A , A 1 , A 2 ), this CI cannot be defined in the quantum case. Another example of that is illustrated below for the IC scenario. Furthermore, because terms such as H ( A , A 1 , A 2 ) are not part of our description, we need, together with the CIs implied by the quantum causal structure, a rule telling us how to relate the entropies of underlying quantum systems to the entropies of their classical descendants, for example, how to relate H ( A 1 , A 2 )→ H ( A ). This is achieved by the data processing (DP) inequality, another basic property that is valid both for the classical and quantum cases [22] . The DP inequality basically states that the information content of a system cannot be increased by acting locally on it. To exemplify, one DP inequality implied by the DAG in Fig. 1 is given by I ( A : B )≤ I ( A 1 , A 2 : B 1 , B 2 ), that is, the mutual information between the classical variables cannot be larger then the information shared by their underlying quantum parents. Defined by the marginal scenario of interest, the third step of the algorithm is identical to the classical case, that is, the elimination of variables representing unobservable random variables or quantum systems. In two of the examples below (IC and quantum networks), all the observable quantities correspond to classical variables, corresponding, for example, to the outcomes of measurements performed on quantum states. Therefore, the marginal description will be given in terms of linear inequalities involving Shannon entropies only. This contrasts with another example we will mention: a generalization of super-dense coding. There, the final description does involve a quantum system, and therefore a mixed inequality with Shannon as well as von Neumann entropy terms results. Information causality The ‘no-signalling principle’ alone is insufficient to explain the ‘degree of non-locality’ exhibited by quantum mechanics [31] . This has motivated the search for stronger, operationally motivated principles, that may single out quantum–mechanical correlations [20] , [32] , [33] , [34] , [35] , [36] , [37] , [38] , [39] . One of these is IC principle [20] , which can be understood as a game: Alice receives a bit string x of length n , while Bob receives a random number s (1≤ s ≤ n ). Bob’s task is to make a guess Y s about the s th bit of the bit string x using as resources a m -bit message M sent to him by Alice and some correlations shared between them. It would be expected that the amount of information available to Bob about x should be bounded by the amount of information contained in the message, that is, H ( M ). IC makes this notion precise, stating that the following inequality is valid in quantum theory [20] where I ( X : Y ) is the classical mutual information between the variables X and Y and the input bits of Alice are assumed to be independent. This inequality is valid for quantum correlations but is violated by all nonlocal correlations beyond Tsirelson’s bound, as originally shown in ref. 20 and further explored in refs 29 , 30 , 40 , 41 . Consider the case where X =( X 1 , X 2 ) is a 2-bit string. The corresponding causal structure to the IC game is the one shown in Fig. 1b ). The only relevant CI is given by I ( X 1 , X 2 : AB )=0. Note that classically the CIs I ( X 1 , X 2 : Y s | M , B )=0 (with s =1, 2) would also be part of our entropic description. However, because we cannot assign a joint entropy to Y s and ϱ B , this classically valid CI cannot be part of the entropic description in the quantum case. We can now proceed with the general framework. But before doing that, we first need to specify in which marginal scenario we are interested. In ref. 20 , the authors implicitly restricted their attention to the marginal scenario defined by { X 1 , Y 1 }, { X 2 , Y 2 }, { M }. Proceeding with this marginal scenario, we find that the only non-trivial inequality characterizing this marginal entropic cone is given by which corresponds exactly to the IC inequality obtained in ref. 30 , where the input bits are not assumed to be independent. Note, however, that using the aforementioned marginal scenario, available information is being discarded. The most general possible marginal scenario is given by { X 1 , X 2 , Y s , M } (with s =1, 2). That is, in this case we are also interested in how much information the guess Y 1 of the bit X 1 , together with the message M , may contain about the bit X 2 (similarly for B 2 and X 1 ). Proceeding with this marginal scenario, we find different classes of non-trivial tight inequalities describing the marginal information causality cone. Of particular relevance is the following tighter version of the original IC inequality Two different interpretations can be given to this inequality: as a monogamy of correlations or as a classical quantification of causal influence. For the first interpretation, consider for simplicity the case where the input bits are independent, that is, I ( X 1 : X 2 )=0. These independent variables may, however, become correlated conditioned on other variables that depend on them. That is, in general I ( X 1 : X 2 | Y 2 , M )≠0. However, the underlying causal relationships between the variables impose constraints on how much we can correlate these variables. In fact, as we can see from (8), the more information the message M and the guess Y i contain about about the input bit X i , the smaller is the correlation we can generate between the input bits by conditioning on them. As an extreme example suppose Alice decides to send M = X 1 ⊕ X 2 . Then X 1 and X 2 are fully correlated given M , but M does not contain any information about the individual inputs X 1 and X 2 . As for the second interpretation, we need to rely on the classical concept of how to quantify causal influence between two sets of variables X and Y . As shown in ref. 42 , a good measure of the causal influence of a variable X over a variable Y should be lower bounded as , where stands for all the parents of Y but X . That is, excluding the correlations between X and Y that are mediated via , the remaining correlations give a lower bound to the direct causal influence between the variables. Consider for instance that we allow for an arrow between the input bits X and the guess Y . Therefore, the classical CI I ( X 1 , X 2 : Y 1 , Y 2 | M , B )=0 that is valid for the DAG in Fig. 1b ), does not hold any longer. In this case , an object that is part of the entropic description in the classical case. Proceeding with the general framework one can prove that That is, the degree of violation of (8) (for example, via a Popescu-Rohrlich(PR)-box) gives a lower bound to the minimum amount of direct causal influence required to obtain the same level of correlations within a classical model. Inequality (8) refers to the particular case of two input bits for Alice. As we prove in the Methods section, the following generalization is valid within the quantum theory for any number of input bits: We further notice that the IC scenario is quite similar to the super-dense coding set-up [21] , where, however, in the latter case the message M is quantum. On the level of the entropies, this difference is manifested by the fact that monotonicity H ( M | X 0 , X 1 , B )≥0 must be replaced by weak monotonicity H ( M | X 0 , X 1 , B )+ H ( M )≥0. As proved in the Methods section, this implies that a similar inequality to (10) is a also valid for the super-dense coding scenario if one replaces the Shannon entropy H ( M ) by twice the von Neumann entropy 2 H ( M ). This generalizes the well-known phenomenon of super-dense coding [21] , which states that in the presence of shared entanglement, the exchange of one d -level system allows for one of d 2 -diferent messages to be communicated. Finally, to understand how much more powerful inequality (8) may be as a witness of post-quantum correlations, we perform a similar analysis to the one in ref. 43 . We consider the following section of the non-signalling polytope with p PR ( a , b | x , y )=(1/2) δ a ⊕ b , xy , p white ( a , b | x , y )=1/4 and p det ( a , b | x , y )= δ a ,0 δ b ,0 corresponding, respectively, to the PR-box, white noise and a deterministic box. The results are displayed in Fig. 2 , where it can be seen that the new inequality is considerably more powerful then the original one. Our new inequality can witness, already on the single-copy level, the postquantumness of distributions that could not be detected before even in the limit of many copies. 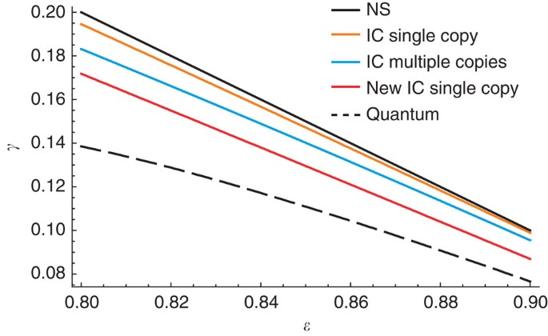Figure 2: Comparison of the strengthened and original IC principles. A slice of the non-signalling polytope corresponding to the distribution (11). The lower black-dashed line is an upper limit on quantum correlations obtained via the criterion in ref.48while the upper solid black line bounds the set of non-signalling correlations. The solid red, blue and orange curves correspond, respectively, to the boundaries obtained with the IC inequalities (8), (6) and (7). Above each of the curves, the corresponding inequalities are violated. SeeSupplementary Note 1for details of how the curves are computed. Figure 2: Comparison of the strengthened and original IC principles. A slice of the non-signalling polytope corresponding to the distribution (11). The lower black-dashed line is an upper limit on quantum correlations obtained via the criterion in ref. 48 while the upper solid black line bounds the set of non-signalling correlations. The solid red, blue and orange curves correspond, respectively, to the boundaries obtained with the IC inequalities (8), (6) and (7). Above each of the curves, the corresponding inequalities are violated. See Supplementary Note 1 for details of how the curves are computed. Full size image Quantum networks Quantum networks are ubiquitous in quantum information. The basic scenario consists of a collection of entangled states that are distributed among several spatially separated parties to perform some informational task, for example, entanglement percolation [17] , entanglement swapping [44] or distributed computing [15] , [16] . A similar set-up is of relevance in classical causal inference, namely the inference of latent common ancestors [14] , [45] . As we will show next, just the topology of these quantum networks already imply non-trivial constraints on the correlations that can be obtained between the different parties. We will consider the particular case where all the parties can be connected by at most bipartite states. We note, however, that our framework applies as well to the most general case and results along this line are presented in the Supplementary Notes 2 and 3 . The problem can be restated as follows. Consider n observable variables that may be assumed to have no direct causal influence on each other (as they are space-like separated). Given some observed correlations between them, the basic question is then: can the correlations between these n variables be explained by (hidden) common ancestors each connecting at most two of them? The simplest of such common ancestors scenarios ( n =3), the so-called triangle scenario [5] , [45] , [46] , is illustrated in Fig. 1a . In the case where the underlying hidden variables are classical (for example, separable states), the entropic marginal cone associated with this DAG has been completely characterized in ref. 7 . Following the framework delineated before, we can prove that facets of this cone are also obtained if we replace the underlying classical variables by quantum states ( Supplementary Note 2 ). This implies that entropically quantum correlations respect the same type of monogamy relations as classical variables. The natural question is how to generalize this result to more general common ancestor structures for arbitrary n . With this aim, we prove in the Methods section that the monogamy relation recently derived in ref. 14 is also valid for quantum theory. We also prove in the Supplementary Note 3 that this inequality is valid for general non-signalling theories, generalizing the result obtained in ref. 9 for n =3. In addition, we exhibit that for any non-trivial common ancestor structure there are entropic constraints even if we allow for general non-signalling theories. The inequality (12) can be seen as a kind of monogamy of correlations. Consider for instance the case n =3 and label the common ancestors (any non-signalling resource) connecting variables V i and V j by ϱ i , j . If the correlation between V 1 and V 2 is large, that means that V 1 has a strong causal dependence on their common mutual ancestor ϱ 1,2 . That implies that V 1 should depend only mildly on its ancestor ϱ 1,3 and therefore its correlation with V 3 should also be small. The inequality (12) makes this intuition precise. In this work, we have introduced a systematic algorithm for computing information–theoretic constraints arising from quantum causal structures. Moreover, we have demonstrated the versatility of the framework by applying it to a set of diverse examples from quantum foundations, quantum communication and the analysis of distributed architectures. In particular, our framework readily allows us to obtain a much stronger version of information causality. These examples aside, we believe that the main contribution of this work is to highlight the power of systematically analysing entropic marginals. A number of future directions for research immediately suggests themselves. In particular, it will likely be fruitful to consider multipartite versions of information causality or other information–theoretical principles and to further look into the operational meaning of entropy inequality violations. A linear programme framework for entropic inequalities Given the inequality description of the entropic cone describing a causal structure, to obtain the description of an associated marginal scenario we need to eliminate from the set of inequalities all variables not contained in . After this elimination procedure, we obtain a new set of linear inequalities, constraints that correspond to facets of a convex cone, more precisely the marginal entropic cone characterizing the compatibility region of a certain causal structure [7] . This can be achieved via a FM elimination, a standard linear programming algorithm for eliminating variables from systems of inequalities [47] . The problem with the FM elimination is that it is a doubly exponential algorithm in the number of variables to be eliminated. As the number of variables in the causal structure of interest increases, typically this elimination becomes computationally intractable. While it can be computationally very demanding to obtain the full description of a marginal cone, to check whether a given candidate inequality is respected by a causal structure is relatively easy. More precisely, the algorithm is admittedly exponential in the number of random variables/quantum systems, but in comparison the FM elimination method for finding all the inequalities is doubly exponential in the number of variables participating in the set of linear inequalities, that is, triply exponential in the number of random variables/quantum systems. Consider that a given causal structure leads to a number N of possible entropies. These are organized in a n -dimensional vector h . In the purely classical case, the graph consisting of n nodes ( X 1 , …, X n ) will lead to a N =2 n -dimensional entropy vector that can be organized as h =( H ( φ ), H ( X n ), H ( X n −1 ), H ( X n −1 X n ), …, H ( X 1 , …, X n )). In the quantum case, since not all subsets of variables may jointly coexist we will have typically that N is strictly smaller than 2 n . As explained in detail in the main text, for this entropy vector to be compatible with a given causal structure, a set of linear constraints must be fulfilled. These linear constraints can be cast as a system of inequalities of the form M h ≥ 0 , where M is a m × N matrix with m being the number of inequalities characterizing the causal structure. Given the entropy vector h , any entropic-linear inequality can be written simply as the inner product , where is the associated vector to the inequality. A sufficient condition for a given inequality to be valid for a given causal structure is that the associated set of inequalities M h ≥ 0 be true for any entropy vector h . That is, to check the validity of a test inequality, one simply needs to solve the following linear programme: In general, this linear programme only provides a sufficient but not necessary condition for the validity of an inequality. The reason for that is the existence of non-Shannon type inequalities, which are briefly discussed in the Supplementary Note 2 . Proving the new IC inequality We provide in the following an analytical proof of the validity of the generalized IC inequality (10) for the quantum causal structure in Fig. 1b ). Further details can be found in the Supplementary Note 1 . Proof: first rewrite the following conditional mutual information as The left-hand side of the inequality (10) can then be rewritten as This quantity can be upper bounded as leading exactly to the inequality (10). In the proof above we have used consecutively (i) the DP inequalities I ( X 1 : Y 1 , M )≤ I ( X 1 : B , M ) and I ( X i : X 1 , Y i , M )≤ I ( X i : X 1 , B , M ), (ii) the fact that (as can be easily proved inductively using the strong subadditivity property of entropies), (iii) the monotonicity H ( M | X 1 , …, X n , B )≥0, (iv) the independence relation I ( X 1 , …, X n : B )=0 and (v) the positivity of the mutual information I ( B : M )≥0. This concludes the proof. Note that this proof can be easily adapted to the case where the message M sent from Alice to Bob is a quantum state. In this case there are two differences. First, because the message is disturbed to create the guess Y i , we cannot assign an entropy to M and Y i simultaneously. That is, in the left-hand side of the inequality (10), we replace I ( X i : Y i , M )→ I ( X i : Y i ) and I ( X 1 : X i | Y i , M )→ I ( X 1 : X i | Y i ). The second difference is in step iii, because we have used the monotonicity H ( M | X 1 , …, X n , B )≥0 that is not valid for a quantum message. Instead of that, we can use a weak monotonicity inequality, namely H ( M | X 1 , …, X n , B )+ H ( M )≥0. Therefore, in the final inequality (10), I ( X i : Y i , M )→ I ( X i : Y i ) and I ( X 1 : X i | Y i , M )→ I ( X 1 : X i | Y i ) and H ( M ) is replaced by 2 H ( M )—where H now stands for the von Neumann entropy. Proving the monogamy relations of quantum networks In the following, we provide an analytical proof of the monogamy inequality (12) in the main text. Further details can be found in the Supplementary Note 2 . We start with the case n =3. For a Hilbert space , we denote the set of quantum states, that is, the set of positive semidefinite operators with trace one, on it by . Theorem 1. Let be a six-partite quantum state on . Let further be an arbitrary measurement for N = A , B , C . Then Proof: DP yields Then we exploit the chain rule twice and afterward DP again, where in the last step, we have used the independence relation between the quantum states. We have therefore for which the right-hand side can be bounded as leading to inequality (22). In the third line of (26) we used strong subadditivity, and in the last line we used that the entropy of a classical state conditioned on a quantum state is positive. This concludes the proof. This proof can easily be generalized to the case of an arbitrary number of random variables resulting from a classical-quantum Bayesian network in which each parent has at most two children. Corollary. 2 Let be an n ( n −1)-partite quantum state on and let be an arbitrary measurement for i =1, ..., n . Then Proof: First, utilize the independences in the same way as in the proof of Theorem 1 to conclude Now continue by induction. For n =3 we have, according to the proof of Theorem 1, Now assume Using the proof of Theorem 1 again and stopping before the last inequality in (26) we get that is, we get where we defined the primed systems by , observing that this yields a classical-quantum bayesian network with n −1 nodes and connectivity two and used the induction hypothesis. This concludes the proof. How to cite this article: Chaves, R. et al . Information–theoretic implications of quantum causal structures. Nat. Commun. 6:5766 doi: 10.1038/ncomms6766 (2015).